The phase diagram of high-pressure superionic ice Superionic ice is a special group of ice phases at high temperature and pressure, which may exist in ice-rich planets and exoplanets. In superionic ice liquid hydrogen coexists with a crystalline oxygen sublattice. At high pressures, the properties of superionic ice are largely unknown. Here we report evidence that from 280 GPa to 1.3 TPa, there are several competing phases within the close-packed oxygen sublattice. At even higher pressure, the close-packed structure of the oxygen sublattice becomes unstable to a new unusual superionic phase in which the oxygen sublattice takes the P2 1 /c symmetry. We also discover that higher pressure phases have lower transition temperatures. The diffusive hydrogen in the P2 1 /c superionic phase shows strong anisotropic behaviour and forms a quasi-two-dimensional liquid. The ionic conductivity changes abruptly in the solid to close-packed superionic phase transition, but continuously in the solid to P2 1 /c superionic phase transition. Several simulation studies indicate that solid Ice-X at pressure >50 GPa, as the temperature is increased to 1,500–2,000 K, will dissociate into a superionic (SI) phase [1] , [2] , [3] , [4] . In this phase, while the oxygens remain on the sites of a body-centred cubic (BCC) lattice, the hydrogens melt and become fully diffusive. Experiments support the simulation results finding significant ionic conductivity in ice at pressures within 50–60 GPa and temperature >750 K (ref. 5 ). More recently, there has been numerical evidence for a transition to a SI phase with an face-centred cubic (FCC) oxygen sublattice at ∼ 100 GPa (ref. 6 ); this study suggested that the FCC-SI phase is stable up to 4 TPa. Besides the interesting physics in this new phase, theoretical studies suggest that SI ice may exist in the mantle of large planets such as Uranus and Neptune as well as exoplanets. In fact, quantitive details of SI ice may influence the understanding of the unusual non-dipolar, non-axisymmetric magnetic fields in Uranus and Neptune [1] , [7] , [8] . Studying SI ice experimentally is difficult. A static diamond anvil cell can generate accurate data however, to date, experiments have trouble reaching pressures beyond 210 GPa (refs 9 , 10 , 11 , 12 ). Shock wave experiments can access higher pressures [13] , but heat the sample significantly. Dynamic ramp compression techniques are a promising approach to reach high pressures at relatively low temperatures [14] , [15] , but so far there are no experimental results that can reach the extremely high pressures of planetary interiors. Because of the experimental difficulties, many studies on high-pressure ice are based on first principle calculations. In the past, several groups reported new ice structures at zero temperature and pressures >50 GPa (refs 16 , 17 , 18 , 19 , 20 , 21 ). These groups have suggested a complex sequence of stable phases as one increases pressure with aspects such as the zero-point energy (ZPE) affecting the relative stability significantly. A recent result, which includes the contribution of the harmonic ZPE [17] , is shown in Fig. 1 . While there are many different phases at zero temperature and they have been subject to constant revision, knowledge about the high-temperature phases has been more limited. BCC-SI and FCC-SI phases have been suggested to be present [2] , [6] . It is interesting to note that the BCC-SI phase has the same oxygen sublattice as its zero-temperature counterpart Ice-X. However, this is not the case for the FCC-SI phase. More than four different zero-temperature structures with lower symmetry than FCC were reported in the pressure range of the FCC-SI phase [6] , [17] . The difference between the BCC-SI and FCC-SI phases raises the question of alternative finite-temperature oxygen sublattices. 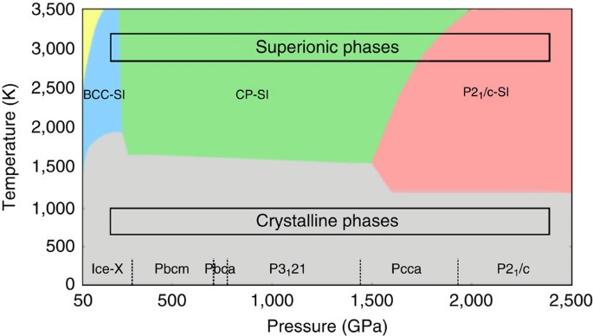Figure 1: Schematic phase diagram of SI ice from 50 GPa to 2.5 TPa. The blue, green and pink regions indicate the three SI phases. The grey region indicates the crystalline regime. The yellow region represents the ionic liquid water phase2. The zero-temperature structures are taken from ref.17. The pressure range of the static structures is consistent with the SI phase diagram, as discussed in the text. SeeSupplementary Fig. 2for more details. Figure 1: Schematic phase diagram of SI ice from 50 GPa to 2.5 TPa. The blue, green and pink regions indicate the three SI phases. The grey region indicates the crystalline regime. The yellow region represents the ionic liquid water phase [2] . The zero-temperature structures are taken from ref. 17 . The pressure range of the static structures is consistent with the SI phase diagram, as discussed in the text. See Supplementary Fig. 2 for more details. Full size image Here we report a comprehensive phase diagram of SI ice ( Fig. 1 ), with the numerical evidence for a new SI phase that is more stable than the FCC-SI phase at pressures >1.6 TPa and which stays stable up to the highest pressures we consider (≈2.5 TPa). This new phase, which we call the P2 1 /c-SI phase, has the P2 1 /c monoclinic oxygen sublattice that is similar to the zero-temperature counterparts P2 1 and P2 1 /c (refs 16 , 17 ). We also suggest evidence that other less symmetrical close-packed structures such as double hexagonal close-packed (dHCP) may be competitive with the FCC-SI phase. We discover that higher pressure phases have lower transition temperatures. In addition, we measure the diffusivity and conductivity in these phases. The diffusive hydrogen in the P2 1 /c-SI phase shows strong anisotropic behaviour and forms a quasi two-dimensional (2D) liquid. The sites occupied most frequently by the diffusing hydrogen do not coincide with the equilibrium sites in the crystalline regime, which indicates strong anharmonicity. The study of the variation of the conductivity with temperature indicates a very different nature of the solid to FCC-SI transition compared with the solid to P2 1 /c-SI transition. We find the ionic conductivity changes abruptly across the solid to FCC-SI phase boundary, while it changes continuously across the solid to P2 1 /c-SI phase boundary. Phase diagram We use constant-pressure ( NPT ) ab-initio molecular dynamics (AIMD) [22] to systematically investigate the SI phase diagram of heavy ice (D 2 O) from 200 GPa to 2.5 TPa. In the classical limit, D 2 O has the same static properties as H 2 O and thus we use H and D interchangeably. We apply the constant-pressure Parrinello–Rahman dynamics that allows the volume and the shape of the cell to vary with time [23] . The new predicted phase diagram is shown schematically in Fig. 1 . In the simulations, we prepare a BCC-SI phase at 200 GPa and 2,200 K as our initial state. This temperature is high enough to keep the system in the SI phase in the pressure range that we cover. The pressure is increased in increments of 40 GPa from 200 GPa to 400 GPa, and increased in increments of 100 GPa from 400 GPa to 1.3 TPa. Given the high diffusivity of the deuterium, the system reaches equilibrium rapidly; the potential energy of the system converges in <0.2 ps. At each step we wait for at least 1 ps to ensure equilibration. At 1.3 TPa, the size of the reference cell is almost twice as big as the real simulation box. For reasons of computational efficiency, we restart our simulation at 1.3 TPa and 1,900 K with a smaller reference box. This simulation starts from the FCC-SI phase, which was suggested to be the most stable phase under this thermodynamic condition [6] . We increase 100 GPa each time from 1.3 TPa to 2.5 TPa and wait at least 2 ps to equilibrate at each step. Owing to the kinetic effects, NPT -AIMD may skip some intermediate phases [24] . Therefore, we also explore the SI phase with different initial conditions to check for any intermediate states. We initialize our system to dHCP, which is a competing phase with FCC, as well as many of the previously suggested zero-temperature structures at different pressures including Pbcm, P3 1 21 and Pcca [17] . We then heat the system at a fixed pressure until the hydrogen sublattice melts. The equilibrium phase boundary between different SI phases and between the solid and SI phases are estimated via single-phase simulations: we vary either the temperature or the pressure such that the system can transform from one structure to another reversibly, while keeping the other thermodynamic variables fixed. For any transition state, there is a pressure and a temperature , the uncertainty of which results from hysteresis effects. Our use of a flexible cell method minimizes the effects of hysteresis allowing for a more accurate identification of phase boundaries. In addition, the fully ionized nature of the SI phase helps attenuate potential difficulties with predicting the right stochiometry and resolving ergodicity issues, which might hamper potential phase separation (stoichiometries different from H 2 O were predicted in ref. 17 to occur at pressure >5 TPa using the ab-initio random structure searching method [25] ). At 2,200 K, we find a reversible transition from the BCC-SI phase to a SI phase with the close-packed oxygen sublattice at [220 GPa, 280 GPa]. This transition pressure does not change appreciably at different temperatures. We find the transition pressure is [200 GPa, 260 GPa] at 3,000 K. The pressure we find is close to the transition pressure from Ice-X to Pbcm [26] at 0 K. This transition was also considered in ref. 6 via free energy calculations where, at 3,000 K, the free energy calculation gave a significantly lower transition pressure at around 100 GPa. At pressures >280 GPa, we find that other less symmetrical close-packed structures may be competitive with the FCC-SI phase: the oxygen sublattice can interconvert between different close-packed structures, which include HCP (AB), dHCP (ABAC), complex-HCP (ABABCACABCBC) and FCC (ABC). The characters in the aforementioned parentheses indicate the stacking layer sequence of each structure, which is the only difference. Since these close-packed structures are very similar and can transform from one structure to another in our simulations, we are not able to distinguish their relative stability. For that reason, we do not distinguish different close-packed structures and refer to this SI phase as the close-packed SI phase (CP-SI). At 1.6 TPa and 1,900 K, the CP sublattice becomes mechanically unstable and it changes to a new SI phase, which we call the P2 1 /c-SI phase. In the P2 1 /c-SI phase, the oxygen sublattice has P2 1 /c symmetry with four atoms in the unit cell. As shown in Supplementary Fig. 1 , this oxygen sublattice is close to the oxygen sublattice in the zero-temperature P2 1 or P2 1 /c structures, which have, however, lower symmetry. In the zero-temperature P2 1 /c structure there are eight O atoms in the unit cell, while the zero-temperature P2 1 structure has four O atoms in the unit cell but lacks the glide plane symmetry of the P2 1 /c structure. Table 1 summarizes the structural parameters of P2 1 /c-SI phase. We also estimate the lower bound of the transition pressure, which is around 1.4 TPa by running the reverse process. Supplementary Fig. 2b summarizes the reversible process we performed. It is interesting to note that the reversible process returns to dHCP but not FCC. At 1,900 K, the P2 1 /c-SI phase is stable up to the highest pressure we consider. The simulations starting from the dHCP and other zero-temperature structures also converge to either the CP-SI phase or the P2 1 /c-SI phase we find after the hydrogen sublattice melts. The details of the simulation results can be found in Supplementary Fig. 2a . Table 1 Structural parameters of the oxygen sublattice of P2 1 /c-SI. Full size table At 1.7 TPa and 1.9 TPa, we locate the transition temperature between the FCC-SI and the P2 1 /c-SI phase as [2,700 K, 3,000 K] and [3,200 K, 3,500 K], respectively. In addition, we estimate the melting temperature of the hydrogen sublattice. As we will discuss later, the solid to FCC-SI phase transition has a sharp change in the conductivity at the melting temperature and thus we can use the conductivity to locate the transition temperature. However, the conductivity changes gradually in the solid to P2 1 /c-SI phase transition. Therefore, it is not straightforward to locate a transition temperature. For that reason, we use a few order parameters, including the maximum peak value of the structure factor and a translational order metric [27] , to locate approximately the transition temperature. These order parameters consistently show that at 1.9 TPa, the transition occurs in the temperature interval [1,100 K, 1,300 K]. See the section on Methods for additional details. Previous theoretical studies showed that the melting temperature of H sublattice is around 1,500 K at 50 GPa (refs 2 , 28 ) and then it rapidly increases to around 2,000 K at [100 GPa, 200 GPa]. At above 200 GPa, we find that though the melting temperature is roughly a constant within the same oxygen sublattice, the melting temperature changes when the oxygen sublattice changes. The melting temperature decreases from 2,000 K to 1,700 K when the oxygen sublattice changes from the BCC-SI to the CP-SI structure, and further decreases to 1,200 K when it changes to the P2 1 /c-SI. When we cool down the system from the SI phases, we find that the frozen crystalline structures are in agreement with previously found zero-temperature structures. In particular, starting from the CP-SI phase at 1.3 TPa and the P2 1 /c-SI phase at 1.9 TPa, the system freezes into static P3 1 21 and P2 1 structures, respectively. Supplementary Fig. 3 shows the comparison of the OH and OO pair correlation functions and coordination number between the quenched structures and zero-temperature structures. Electronic structure We examine the electronic structure in the SI phase. Previous simulations indicated that at 0 K, the highly compressed ice behaves like a network of highly compressed oxide ions [16] . We find a similar behaviour in the P2 1 /c-SI phase. The SI phase is ionically conducting but electronically insulating. Thus, we can characterize its valence electronic structure in terms of maximally localized Wannier functions [29] . In particular it is interesting to plot the distribution of distances between each maximally localized Wannier center (MLWC) and the nearest O atom, as shown in Fig. 2 . This shows a unimodal distribution, very different from the bimodal distribution observed in liquid water or ice at standard pressure conditions [30] , which shows donor and acceptor hydrogen bonds (H-bonds). 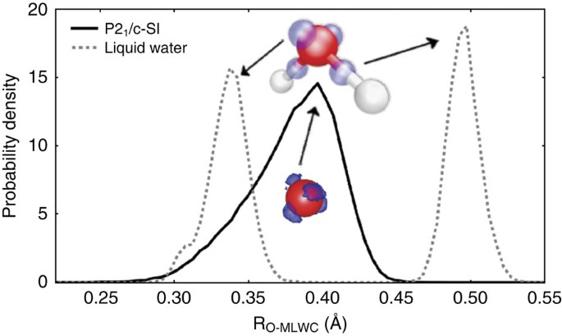Figure 2: Radial distribution function of MLWC. The cartoon shows the distribution of the MLWC (depicted in blue) in real space. The red and silver balls are the oxygen and hydrogen atoms, respectively. The MLWC distribution and atom position from a liquid water simulation at standard temperature and density30is also shown for comparison (paler colours and dashed line). The dramatic change in the MLWC distribution signals a dramatic change in the chemical bond from low to high pressure phases of water (see text). Figure 2 also reports the distribution of the MLWC in real space. The MLWC distribute tetrahedrally around O, which is in agreement with a nominal O 2− charge state [31] . The dramatic change in the MLWC distribution of SI ice relative to standard water signals a dramatic change in the nature of the chemical bond: at high pressure ionic bonds replace the H-bonds between molecular units that characterize the low pressure phases of water. Figure 2: Radial distribution function of MLWC. The cartoon shows the distribution of the MLWC (depicted in blue) in real space. The red and silver balls are the oxygen and hydrogen atoms, respectively. The MLWC distribution and atom position from a liquid water simulation at standard temperature and density [30] is also shown for comparison (paler colours and dashed line). The dramatic change in the MLWC distribution signals a dramatic change in the chemical bond from low to high pressure phases of water (see text). Full size image In the condensed phase, the nominal ionic charges are ill-defined. On the other hand, dynamical Born charges, which represents the response of the system to a perturbation, are well-defined for an electronically insulating system like SI ice. We calculate the dynamical Born charge tensors Z * i , αβ for a large number ( ∼ 100) of snapshots along the dynamical trajectories. We use the electric enthalpy method [32] , which gives , where ∂ F i , α is the change of atomic force in direction α on ion i due to an homogeneous electric field ∂ E β applied in direction β . Following ref. 33 , we analyse the charge tensor in terms of isotropic and anisotropic components, see Supplementary Table 1 and Supplementary Note 1 for more details. In the CP-SI and P2 1 /c-SI phases we find the average isotropic component are +(1.2±0.1) and −(2.4±0.2) for deuterium and oxygen ions, respectively. The corresponding values in the BCC-SI phase are +(1.0±0.1) and −(2.0±0.2). The small difference from the nominal values indicates a contribution due to the electronic response. The average isotropic components of the effective charges are the same at different snapshots and do not change appreciably in the zero-temperature counterparts, which indicates that the electronic structure does not change appreciably across the transition. Ionic transport In our simulations, the diffusion coefficient of the cations is readily calculated by monitoring their mean square displacement (MSD) or by integrating their velocity autocorrelation function. Unlike the BCC-SI or CP-SI phase, the P2 1 /c-SI has a monoclinic structure and it shows a large anisotropic effect in the diffusion coefficient tensor. Using the velocity autocorrelation function, we identify the principle diffusion axes along [201], [010] and [201] × [010] of the P2 1 /c-SI. At 1.9 TPa and 1,600 K, the diffusion coefficient ratio among these three axes is roughly 4:3:1. Thus, the primary diffusion happens in a quasi 2D layer, as shown in Fig. 3 . Hermann et al. [34] suggested a diffusion path in the P2 1 crystalline structure at 0 K via the nudged elastic band method. It is interesting to note that the most diffusive path at finite temperature is not following the lowest energy path at 0 K. The transition path they found is along the [100] direction in the P2 1 /c-SI, which forms an angle of ∼ 30° with the 2D diffusion layer. In the unit cell of P2 1 /c-SI, there are six out of eight hydrogen ions in the quasi 2D diffusion layer, but the other two hydrogen ions are more localized. In the 2D diffusion layer there are four ‘sausage’-like high density regions which are indicated by the green lines in Fig. 3 . These four ‘sausages’ are indistinguishable in the P2 1 /c-SI phase. However, when the system freezes into the crystalline phase, two of the sausages are occupied by two hydrogen ions, while the other two only contain one hydrogen ion that stays in the centre of the sausage, as shown in panel ( c ) of Fig. 3 . The fact that the most frequently occupied sites at high temperature do not coincide with the crystalline sites indicates strong anharmonicity. 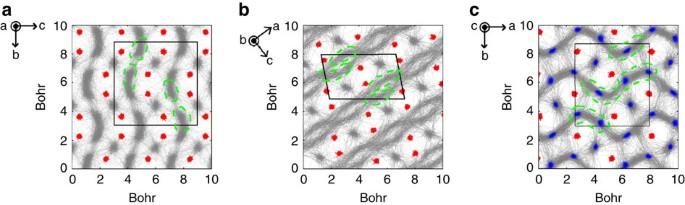Figure 3: Traces of the trajectories of D and O ions. The traces of the trajectories are accumulated over 8 ps in the P21/c-SI at 1,400 K and 1.9 TPa. The red and grey regions are traces of the trajectories of each individual O and D ions, respectively. The green dash lines indicate the ‘sausage’-like high density regions of D. The solid black line indicates the unit cell of P21/c-SI. The O ions oscillate around the equilibrium positions, while the D ions are fully diffusive. (a) Projection along [201] of the P21/c-SI unit cell. (b) Projection along [010] of the P21/c-SI unit cell. (c) Projection along [201] × [010] of the P21/c-SI unit cell. The blue regions are traces of the trajectories of D ions at 400 K and 1.9 TPa, when the system is in the crystalline regime. The different distribution of blue and grey traces indicates strong anharmonicity. Figure 3: Traces of the trajectories of D and O ions. The traces of the trajectories are accumulated over 8 ps in the P2 1 /c-SI at 1,400 K and 1.9 TPa. The red and grey regions are traces of the trajectories of each individual O and D ions, respectively. The green dash lines indicate the ‘sausage’-like high density regions of D. The solid black line indicates the unit cell of P2 1 /c-SI. The O ions oscillate around the equilibrium positions, while the D ions are fully diffusive. ( a ) Projection along [201] of the P2 1 /c-SI unit cell. ( b ) Projection along [010] of the P2 1 /c-SI unit cell. ( c ) Projection along [201] × [010] of the P2 1 /c-SI unit cell. The blue regions are traces of the trajectories of D ions at 400 K and 1.9 TPa, when the system is in the crystalline regime. The different distribution of blue and grey traces indicates strong anharmonicity. Full size image Compared with the BCC-SI and CP-SI phases, the average isotropic diffusion coefficient is smaller in the P2 1 /c-SI phase. This is because there are less empty hydrogen sites in P2 1 /c-SI unit cell. We define the hydrogen sites by locations of maximal hydrogen density. 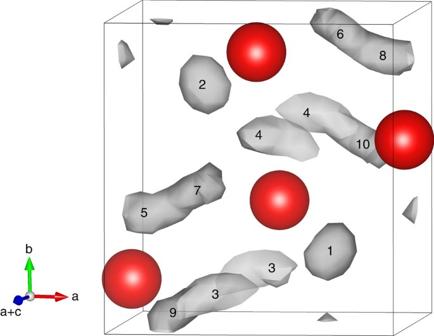Figure 4: Oxygen sublattice and hydrogen density distribution in the P21/c-SI phase. The red balls indicate oxygens and the grey region indicates the distribution of hydrogens. The three axes are along [100] (a), [010] (b) and [101] (a+c). The label from 1 to 10 indicates the density maxima. Site 1 and site 2 are the more localized sites, and the rest are in the diffusion planes. Repeated sites reflect periodicity. Figure 4 shows the isosurface of the density distribution of hydrogens in the P2 1 /c-SI phase. In the unit cell of the P2 1 /c-SI, we find 10 sites with maximal hydrogen density. Among these 10 sites, site 1 and 2 are the localized sites between the diffusion planes and the other 8 of them are located in the diffusion planes (see also Fig. 3 ). The fact that there are only two empty sites in the unit cell makes diffusion slow. Contrast this with the HCP sublattice where there are two empty sites per hydrogen atom. Figure 4: Oxygen sublattice and hydrogen density distribution in the P2 1 /c-SI phase. The red balls indicate oxygens and the grey region indicates the distribution of hydrogens. The three axes are along [100] (a), [010] (b) and [101] (a+c). The label from 1 to 10 indicates the density maxima. Site 1 and site 2 are the more localized sites, and the rest are in the diffusion planes. Repeated sites reflect periodicity. Full size image We estimate the ionic conductivity of heavy ice at 1.3 TPa (FCC) and 1.9 TPa (P2 1 /c), and from 1,100 to 2,500 K via Nernst–Einstein relations , where σ D is the average isotropic ionic conductivity, which is defined as one-third of the trace of the conductivity tensor, n D is the density of the mobile ions (D ions), D D is the average isotropic diffusion coefficient of D estimated from the MSD, and is the average isotropic Born effective charge of D. The average ionic conductivities of the SI phases at different thermodynamic conditions are ∼ 90 S cm −1 (BCC-SI, D 2 O, 200 GPa, 2,500 K), ∼ 120 S cm −1 (FCC-SI, D 2 O, 1.3 TPa, 2,000 K) and ∼ 60 S cm −1 (P2 1 /c-SI, D 2 O, 1.9 TPa, 2,500 K). If we replace the D with H, we find the conductivity of H is roughly 1.2–1.3 times of the conductivity of D. The conductivity we find in the BCC-SI phase is in agreement with the result reported by French et al. [35] . The conductivity in the CP-SI phase is higher and that in the P2 1 /c-SI phase is lower than in the BCC-SI phase. In all the three SI phases, however, the conductivity is in the range of the dissociated water phase in the outer shell of Uranus and Neptune (10–120 S cm −1 ) [1] . The similar ionic conductivity of the SI phase and the ionic water in the outer shell of Uranus and Neptune is consistent with the model suggested by Stanley et al. [7] , which assumed equal conductivity across different phases. SI phases can be classified into three types [36] . In type I, the conductivity jumps at the transition temperature, while it gradually transforms in type II and has Arrhenius behaviour in type III. It is interesting to note the different behaviour between the FCC-SI and P2 1 /c-SI (see Fig. 5a for the change of conductivity across the solid to SI phase boundary). The discontinuity of the conductivity in the FCC-SI phase indicates a type-I transition, while the conductivity of the P2 1 /c-SI phase, which behaves similarly to the Ice-X to BCC-SI transition [28] , is more continuous and belongs to type-II transition [36] . Type-I SI transitions are known to be accompanied by a structural transition in the crystalline sublattice, but in type-II SI conductors this structural transition is absent [36] . We observe the same behaviour here. When the hydrogen ions stop moving, the FCC-SI phase freezes into the P3 1 21 phase at 1.3 TPa. These two structures have different oxygen sublattices. On the contrary, despite the different symmetry, the P2 1 /c-SI has a very similar oxygen sublattice to the solid P2 1 /c or P2 1 phase. We confirm this with the MSD of oxygen ions in these two phases, which is shown in Fig. 5b . There is a sudden change of the MSD as we cross the phase boundary between the FCC-SI phase and P3 1 21, while the MSD changes gradually as the phase changes from P2 1 to P2 1 /c-SI. 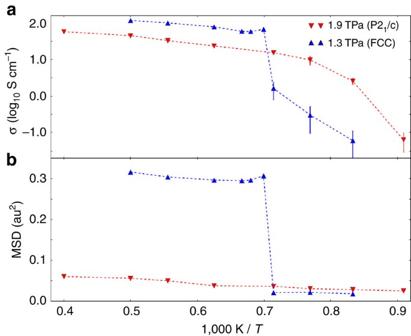Figure 5: Ionic conductivity and MSD of oxygen. (a) Ionic conductivity across the solid to SI phase transition. (b) The MSD of oxygen. The error bars indicate the standard error estimated with three non-overlapping intervals. Error bars smaller than the symbols are not shown in the graph. Notice the sharp change in the MSD in correspondence to the transition from P3121 to FCC-SI. By contrast, the transition from P21(0 K) to P21/c-SI does not show any signature in the MSD. Figure 5: Ionic conductivity and MSD of oxygen. ( a ) Ionic conductivity across the solid to SI phase transition. ( b ) The MSD of oxygen. The error bars indicate the standard error estimated with three non-overlapping intervals. Error bars smaller than the symbols are not shown in the graph. Notice the sharp change in the MSD in correspondence to the transition from P3 1 21 to FCC-SI. By contrast, the transition from P2 1 (0 K) to P2 1 /c-SI does not show any signature in the MSD. Full size image Remarks on nuclear quantum effects In nature, the cations in ice come in two isotopes–hydrogen and deuterium. Classically, any isotope effect manifests itself only in dynamic properties such as the vibrational spectra ( Fig. 6 ), diffusivity and ionic conductivity. Quantum mechanically isotope effects manifest also in static properties. Previous work [17] shows that harmonic ZPE affects significantly the zero-temperature phase diagram of high-pressure ice. Such an effect has also been seen at finite temperature for elemental material systems at high pressure such as Li (ref. 37 ) and H (ref. 38 ). With the possible exception of H at very high pressure, these nuclear quantum effects were found to have only minor corrections on the classically calculated melting lines. Here we estimate the magnitude of this effect in SI ice by looking at the vibrational frequency. Previous studies showed that at 0 K (ref. 34 ), the vibrational frequency in P2 1 can be as high as 5,000 cm −1 for H or 3,000 cm −1 for D. The corresponding ZPE is about 1.28 eV mol −1 for H 2 O or 0.99 eV mol −1 for D 2 O. Using the power spectrum of the velocity autocorrelation function [39] , we show the density of states of the single-particle dynamics in P2 1 /c-SI in Fig. 6 . In comparison with the zero-temperature spectrum, the H (D) ions have a diffusive mode at f =0, and owing to the molten hydrogen sublattice, the highest frequency mode, which is related to the stretching mode along the O–H ionic bond, becomes weaker in the SI phase. We also find a softening of the vibrational modes for the oxygen sublattice in the SI phase. The average vibrational frequency of the oxygen sublattice decreases from 1,580 cm −1 in the zero-temperature P2 1 structure to 1,480 cm −1 in P2 1 /c-SI. The ZPE in the P2 1 /c-SI phase is significantly higher than the energy necessary to melt the H sublattice and it could affect the phase diagram even at the temperature of the SI transition. However, determining the quantum effect requires substantial additional work and is beyond the scope of this paper. 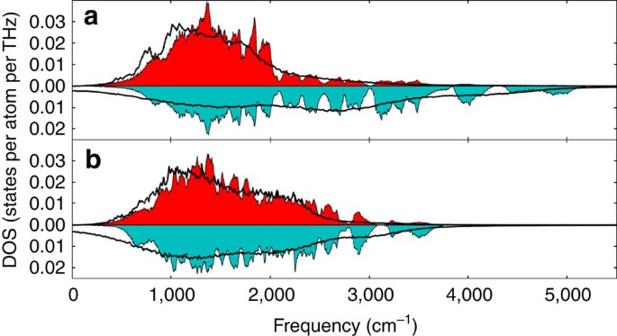Figure 6: Dynamical density of states (DOSs) of crystalline P21and P21/c-SI. (a) DOS of H2O. (b) DOS of D2O. The red and blue areas are the DOS of H/D and O of the zero-temperature P21structure34. The thick dark line on top of it indicates the DOS of the P21/c-SI phase at 2,000 K. The non-zero DOS at zero frequency shows the diffusive nature of H/D in the SI phase. Figure 6: Dynamical density of states (DOSs) of crystalline P2 1 and P2 1 /c-SI. ( a ) DOS of H 2 O. ( b ) DOS of D 2 O. The red and blue areas are the DOS of H/D and O of the zero-temperature P2 1 structure [34] . The thick dark line on top of it indicates the DOS of the P2 1 /c-SI phase at 2,000 K. The non-zero DOS at zero frequency shows the diffusive nature of H/D in the SI phase. Full size image Having identified a new P2 1 /c-SI crystal structure we now ask what drives the transition out of the CP-SI phase. At extremely high pressure, the specific enthalpy is dominated by the product of pressure ( P ) and specific volume ( V ) term, which means that a more stable phase should have a higher density, and thus a larger packing fraction. Although the CP structures are the densest arrangements for a unary system, the presence of hydrogen makes denser structures possible. At 1,900 K and 1.6 TPa, we find a 0.7% volume reduction, or 0.19 Bohr 3 per mol when the oxygen sublattice changed from the CP-SI structure to P2 1 /c-SI. Owing to the higher density, P2 1 /c-SI has a lower enthalpy than CP-SI, and thus it is more stable at higher pressure. Table 2 summarizes the enthalpy difference between FCC-SI and P2 1 /c-SI. When the CP-SI sublattice changes to the P2 1 /c-SI sublattice, the first shell of oxygen neighbours splits into two closely spaced shells. The readjustment of the oxygen positions allows one more oxygen to move closer. Supplementary Fig. 1 shows the O–O pair correlation functions and the coordination number of the oxygen sublattice for the CP-SI and P2 1 /c-SI phase, normalized to the same density. Compared with the CP-SI sublattice, which has 12 neighbours in the first shell, the P2 1 /c-SI sublattice does not have a well separated first and second shell. Instead, each oxygen has 13 neighbours within close distance. If one increases the temperature to ∼ 3,000 K at 1.7 TPa, the P2 1 /c-SI phase transforms back to the CP-SI phase. On the phase boundary at 3,000 K, the P2 1 /c-SI phase still has a lower enthalpy of about 0.1 eV mol −1 . The fact that the P2 1 /c-SI phase spontaneously changes back to the CP-SI phase suggests a larger entropy in the CP-SI phase. This behaviour is consistent with the observed larger diffusivity and hence a larger disorder in the H sublattice of the CP-SI phase. Table 2 Change of thermodynamic properties in the FCC-SI to P2 1 /c-SI transition. Full size table Compared with the zero-temperature stable structures, the SI ice phase diagram in Fig. 1 is significantly simpler. We can understand this as follows. At 0 K, as pressure is increased, the first stable structure after Ice-X is Pbcm [26] , followed by Pbca [18] and by P3 1 21 (ref. 17 ). Although these structures have different H sublattices, they all have a distorted CP O sublattice with the first 12 neighbours well separated from the next 6. In P2 1 /c, a thirteenth O neighbor has moved to close distance. In Pcca the thirteenth neighbor has only moved midway between the first and the second group of neighbours, characteristic of the CP-like structures. Thus Pcca can be seen as an intermediate structure between P3 1 21 and P2 1 /c. In Supplementary Fig. 1 , we give more details to illustrate the systematic change with pressure of the pair correlation function and coordination number of the O sublattice at 0 K. P2 1 and P2 1 /c differ mainly in their H sublattices. Obviously on melting the H sublattice, the differences of the hydrogen sublattice disappear. Without the structure supplied by the extra hydrogen sublattice, the positions of oxygen ions change slightly with slightly different oxygen sublattices converging to a more symmetric structure. It is these more symmetric structures that appear in the SI phases. The phase diagram indicates two additional novel effects. First, there are two crystalline phases that melt on increasing the pressure; this is a result of the monotonic decrease in melting temperature as we move along the sequence BCC-SI→CP-SI→P2 1 /c-SI. Second, the phase diagram has a number of regions where the phase boundary has a negative d T /d P slope. This is true in the transition region between the solid and SI phases where the negative slope must exist if the melting temperature decreases to avoid a SI phase freezing on an increase in temperature. Moreover, we can understand the sign of both these slopes as well as that of the SI to SI slopes using the Clausius–Clapeyron relation d T /d P =Δ V /Δ S , where Δ V and Δ S are the specific volume and entropy change of the phase transition, respectively. The slope of the coexistence line between two phases is negative if the denser phase has higher entropy while it is positive otherwise. Our calculated diffusivities suggest that under the considered thermodynamic conditions the CP-SI phase has higher entropy than either BCC-SI or P2 1 /c-SI. Thus, the slope of the BCC-SI to CP-SI boundary should be negative, while that of the CP-SI to P2 1 /c-SI boundary should be positive, in agreement with our simulation results. Moreover, similar considerations suggest that the solid to CP-SI and the solid to P2 1 /c-SI transitions must be negative slope in the regions of melting temperature drop, as the entropy is likely to increase in a solid to SI transition. Finally, away from the regions where the melting temperature drops sharply ( Fig. 1 ) the almost flat melting curves of CP-SI and of P2 1 /c-SI indicate a small volume change from the underlying solid to SI phases. In summary, we provide a comprehensive SI ice phase diagram from 200 GPa to 2.5 TPa and up to 3,500 K in the classical limit. At 1,900 K, we find a transition between the CP-SI phase and the P2 1 /c-SI phase at 1.4–1.6 TPa. This new SI phase is stable up to at least 2.5 TPa. The melting temperature of the hydrogen sublattice has negative d T /d P slope across the SI phase boundaries, and it decreases when the system changes to a high-pressure SI phase. In all of the SI phases, H and O are highly ionized. We evaluate the ionic conductivity of SI ice and show that the CP-SI and P2 1 /c-SI phases belong to different types of SI phase. We also see a large anisotropic effect in the new SI phase in which the diffusion of hydrogen is mainly in a quasi 2D layer. Owing to fewer hydrogen sites in the 2D plane, P2 1 /c-SI has a smaller diffusion coefficient. Finally, the large vibrational frequencies suggest the nuclear quantum effect in the SI phase could be significant even at the transition temperature. It may affect the phase boundary and need further studies. Constant-pressure AIMD We use the QUANTUM ESPRESSO (ref. 40 ) software package to perform the NPT -AIMD simulations, with the Perdew–Burke–Ernzerhof density functional and norm conserving pseudopotentials [41] , [42] ( http://fpmd.ucdavis.edu/potentials/index.htm ). We check that the adopted pseudopotentials for O and H work at high pressure as discussed in the Supplementary Note 2 . The temperature is controlled by a single Nose–Hoover thermostat. We use gamma point sampling and relatively large simulation boxes containing at least 108 molecules. We carefully check that the relative phase stability does not change when we use more extensive k-point sampling. To use a larger time step, we use the heavy water molecule (D 2 O) in most of our simulations. In the classical limit, D 2 O has the same static properties as H 2 O. We use a plane wave energy cut-off of 1,500 eV, with the effective constant energy cut-off technique [43] , which adjusts the number of plane waves used in the density functional theory (DFT) calculation as the box size and shape changes. It has been shown that the total energy converges faster with constant energy cut-off than with constant number of plane waves [44] . Therefore, when the simulation box changes its shape, it is preferable to keep the energy cut-off constant. In the implementation, the electronic wave function is expanded with a fixed number of plane waves. Each plane wave function has a variable weight that can vary between 1 and 0 to mimic constant energy cut-off. At the beginning, the number of plane waves is determined by a reference cell that is always larger than the real simulation box during the simulation, thus it can cover the Hilbert space up to the energy cut-off. During the simulation, the weight of plane waves that cross the energy cut-off drops rapidly but continuously to zero. To avoid wasting central processing unit time, one should choose the reference cell close to the real simulation box such that the total number of plane waves is not too large compared with the active number. Locating the solid to P2 1 /c-SI phase transition temperature The solid to P2 1 /c-SI transition is a type-II SI phase transition, which does not have a sharp change in the conductivity. Therefore, we are not able to use the conductivity to locate the transition temperature. On the other hand, the structure factor, which is defined as , provides a better means to locate the transition temperature. We use the nonnegative scalar ‘order’ metric τ introduced in ref. 27 , which is defined as , where N is the number of particles, as well as the intensity of S ( k M −600 ), where k M −600 is the wave vector associated with highest peak of S ( k ) at 600 K, to characterize the degree of disorder. For a spatially uncorrelated configuration of particles (ideal gas) in the infinite-volume limit, S ( k )=1 for all k and hence τ takes on its minimum value of zero. When the system is correlated, then S ( k ) will generally deviate from zero, and yield a positive value of τ , providing a measure of the deviation from perfect disorder. 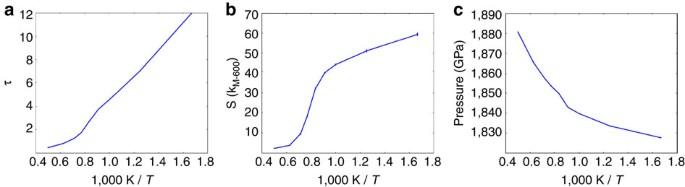Figure 7: Order parameters across the P21to P21/c-SI transition. (a) Variation withTof the order metricτof hydrogen. (b) Variation withTof the highest peak of S(k) of hydrogen. (c) Variation withTof the pressure at fixed specific volume. All three measures indicate a transition temperature in the interval [1,100 K, 1,300 K], or inverse-temperature interval [0.77, 0.91]. Figure 7 shows the two order parameters as a function of temperature at 1.9 TPa. Owing to the finite size of our system, we cannot locate the phase boundary very precisely. However, both of these two order parameters increase relatively rapidly in the temperature range from 1,100 to 1,300 K. In addition, we show that with a fixed simulation box, the pressure as a function of temperature has an inflection point at (1,100 and 1,200 K). Since all of these three quantities consistently show that there is a relatively rapid change in slope in the temperature interval (1,100 and 1,300 K), we conclude at 1.9 TPa the transition temperature is (1,100 and 1,300 K). Figure 7: Order parameters across the P2 1 to P2 1 /c-SI transition. ( a ) Variation with T of the order metric τ of hydrogen. ( b ) Variation with T of the highest peak of S( k ) of hydrogen. ( c ) Variation with T of the pressure at fixed specific volume. All three measures indicate a transition temperature in the interval [1,100 K, 1,300 K], or inverse-temperature interval [0.77, 0.91]. Full size image How to cite this article : Sun, J. et al. The Phase Diagram of High-Pressure Superionic Ice. Nat. Commun. 6:8156 doi: 10.1038/ncomms9156 (2015).